An electrostatic model for the determination of magnetic anisotropy in dysprosium complexes Understanding the anisotropic electronic structure of lanthanide complexes is important in areas as diverse as magnetic resonance imaging, luminescent cell labelling and quantum computing. Here we present an intuitive strategy based on a simple electrostatic method, capable of predicting the magnetic anisotropy of dysprosium(III) complexes, even in low symmetry. The strategy relies only on knowing the X-ray structure of the complex and the well-established observation that, in the absence of high symmetry, the ground state of dysprosium(III) is a doublet quantized along the anisotropy axis with an angular momentum quantum number m J =± 15 / 2 . The magnetic anisotropy axis of 14 low-symmetry monometallic dysprosium(III) complexes computed via high-level ab initio calculations are very well reproduced by our electrostatic model. Furthermore, we show that the magnetic anisotropy is equally well predicted in a selection of low-symmetry polymetallic complexes. The fascinating magnetic properties of the lanthanides have continued to be a highly topical and strongly multi-disciplinary research area for over 60 years. Such is the diversity of this field that their application reaches from magnetic resonance imaging and cell labelling [1] , [2] , to potential building blocks of quantum computers [3] . The pursuit of such applications relies on detailed knowledge of the magnetic anisotropy, which, while being completely defined in cases of high symmetry, is difficult to elucidate in low-symmetry complexes. Much recent work, where 4f complexes have shown slow magnetic relaxation [4] , [5] , [6] , [7] and unprecedented non-collinear magnetic textures at the single-molecule level [8] , [9] , [10] , also depends on understanding the orientation of the magnetic anisotropy. Of all the lanthanide ions, it is Dy III that continues to prove the most interesting, providing unexpected examples of new magnetic phenomena, by virtue of its unique magnetic anisotropy [11] . However, because of the intricate electronic structure of lanthanide complexes, simple models that can predict magnetic anisotropy in molecular solids of low symmetry are still missing. The single-ion properties of 4f metal ions, whether in mono- or polymetallic complexes, are difficult to elucidate owing to the shielded nature of the 4f orbitals giving rise to weak interactions with the surrounding environment. Recent advances in post Hartree-Fock multi-configurational ab initio methodology have made accurate quantum chemical calculations on paramagnetic 4f compounds possible [12] . The Complete Active Space Self Consistent Field (CASSCF) method can accurately predict the magnetic properties of lanthanide complexes [13] , [14] , and calculations of this type have become an indispensable tool for the explanation of increasingly interesting magnetic phenomena [6] , [15] , [16] , [17] . These calculations are especially useful in cases of low symmetry, where previous methods have provided intractable, over parameterized problems [18] , [19] . Although CASSCF ab initio calculations are extremely versatile and implicitly include all effects required to elucidate the magnetic properties, the results offer little in the way of chemically intuitive explanations and to obtain reliable results requires considerable intervention by expert theorists equipped with access to powerful computational resources. Recently, some of us have applied a simple electrostatic model to rationalize the unexpected direction of the calculated magnetic anisotropy in two related sets of monometallic 4f complexes [20] . This was based on the aspherical electron density distributions of the lanthanide ions, pioneered by Sievers [21] , and the design principles for the exploitation of f-element anisotropy outlined by Rinehart and Long [22] . Other groups have also been coming to similar conclusions [17] . Although the use of crystal field methods to model anisotropic magnetic data is widespread [23] , [24] , [25] , models for the prediction of magnetic anisotropy in low symmetry are few [26] , [27] . These methods are based on the diagonalization of a crystal field Hamiltonian, which, especially in cases of low symmetry, requires a large number of parameters that often can only be reliably determined by fitting experimental data. Such an approach can obscure the rationalization of magnetic anisotropy and its predictive power is uncertain. Here we report a quantitative method based on a straightforward electrostatic energy minimization for the prediction of the orientation of the ground state magnetic anisotropy axis of dysprosium(III) ions, which does not rely on the fitting of experimental data, requiring only the determination of an X-ray crystal structure. Many electron wavefunction and electrostatic minimization An increasing number of ab initio CASSCF calculations [6] , [14] , [15] , [20] , [28] have shown that in most low-symmetry complexes, the ground Kramers doublet of Dy III is strongly axial with the principal values of the g -tensor approaching those of the m J =± 15 / 2 levels of the atomic multiplet 6 H 15/2 ( g x = g y =0, g z =20). This empirical observation suggests that a simple, but appropriate, variational ansatz for the many-electron ground state wavefunction of these low-symmetry complexes consists of the atomic functions ψ ± ( α , β ) corresponding to the m J =± 15 / 2 states of the multiplet 6 H 15/2 . The variational parameters to be optimized in ψ ± ( α , β ) consist of the two polar angles α and β , which specify the orientation of the quantization axis with respect to the low-symmetry crystal field V CF defined by the ligands. To determine these angles, and hence the full g -tensor of the ground Kramers doublet of the Dy III complex, we can use the variational principle and minimize the energy with respect to all possible orientations ( α , β ) of the quantization axis. This proposed strategy is readily mapped onto a classical electrostatic energy minimization problem. Following the work of Sievers [21] , the many-electron wavefunctions ψ ±( α , β ) can be described by an electron density distribution , where θ and φ are polar angles defined in the reference frame of V CF , expressing the angular dependence of the axially symmetric aspherical electron density. This aspherical f-electron density can be written as a linear combination of three spherical harmonics Y 2,0 ( θ , φ ), Y 4,0 ( θ , φ ) and Y 6,0 ( θ , φ ), where the coefficients of each are fully determined by angular momentum coupling and average atomic radial multipole moments [21] . In the particular case of Dy III , can be approximated by an oblate spheroid distribution owing to the dominant contribution of the quadrupolar term Y 2,0 ( θ , φ ) to the expansion [22] , [21] . As the crystal field is a one-electron potential, the many-electron variational integral E ±15/2 ( α , β ) can be exactly recast into a simple electrostatic energy integral, describing the interaction between the electric potential generated by the crystal field V CF ( θ , ϕ ) and the Sievers charge density associated with the f-electrons in the central Dy III ion (equation (1)). Thus, we arrive at the hypothesis that in low-symmetry Dy III complexes, the many-electron ground state wavefunction and, hence, the orientation of the magnetic anisotropy axis, can be determined simply by solving a classical electrostatic energy minimization problem. Constructing the crystal field potential of charged ligands To use this hypothesis, we must determine the explicit form of V CF ( θ , ϕ ) appearing in equation (1), by using an appropriate model for the charge distribution on the ligands. This may appear a difficult problem; here, we use a simple model for charged ligands that are common in many low-symmetry Dy III complexes. The charge on the ligands is expected to have a dominant role in the determination of the electrostatic potential experienced by Dy III , and thus, we can calculate the electrostatic field produced by charge on the ligands within a minimal valence bond (VB) model. Within this model, the charge is delocalized as a resonance hybrid that can be seen as a weighted sum of all ‘chemically stable’ Lewis structures ( Fig. 1 ); this is a representation of the leading contribution to the full VB wavefunction. By taking the sum of the partial charges accumulated by each atom in the VB resonance hybrid, q n , we arrive at a very simple fractional charge distribution for the ligand, where, typically, very few atoms will accommodate a charge and most will remain neutral. Our strategy is to construct the crystal field potential solely from the fractional charges determined by the VB resonance hybrid, excluding neutral atoms entirely (see Fig. 1 illustrating the fractional charges of the resonance hybrids for the ligands of interest here). The partitioning of the charge without any need for computation illustrates the elegance of our model. 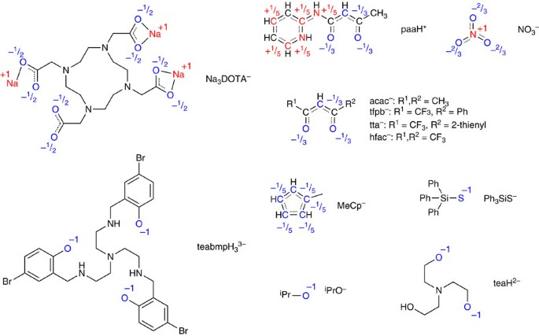Figure 1: Partial charges assigned to the formally charged ligands in complexes 1–17. The zwitterionic N-(2-pyridyl)-acetylacetamide (paaH*) has two formal charges owing to the deprotonation of the α-carbon and protonation of the pyridyl nitrogen. Each pendant carboxylate arm of the macrocyclic trisodium 1,4,7,10-tetraazacyclododecaneN,N′,N′′,N′′′-tetraacetate ligand (Na3DOTA−) has a single negative charge that is delocalized evenly over the two oxygen atoms; three of the four acetate arms bind sodium cations, which each have a single positive charge. The aromatic anion of methylcyclopentadienyl (MeCp−) has a single negative charge that is delocalized evenly over the five cyclic carbon atoms. Not shown: Compounds12and13contain Zn2+ions, which have formal charges of positive two in our model. Compound17contains a central oxide (O2−) ligand, which has a formal charge of negative two in our model. Figure 1: Partial charges assigned to the formally charged ligands in complexes 1–17. The zwitterionic N-(2-pyridyl)-acetylacetamide (paaH*) has two formal charges owing to the deprotonation of the α-carbon and protonation of the pyridyl nitrogen. Each pendant carboxylate arm of the macrocyclic trisodium 1,4,7,10-tetraazacyclododecane N , N ′, N ′′, N ′′′-tetraacetate ligand (Na 3 DOTA − ) has a single negative charge that is delocalized evenly over the two oxygen atoms; three of the four acetate arms bind sodium cations, which each have a single positive charge. The aromatic anion of methylcyclopentadienyl (MeCp − ) has a single negative charge that is delocalized evenly over the five cyclic carbon atoms. Not shown: Compounds 12 and 13 contain Zn 2+ ions, which have formal charges of positive two in our model. Compound 17 contains a central oxide (O 2− ) ligand, which has a formal charge of negative two in our model. Full size image Once the partitioning of the charge over the ligand is determined, the resulting partial charges are arranged around the central Dy III ion using the known X-ray crystal structure of the complex, allowing the electrostatic potential to be easily calculated using crystal field theory [29] (equation (2), where ( R n , θ n , ϕ n ) are the spherical coordinates of the n th charged atom, see Methods section). Minimization of the electrostatic energy in equation (1) in conjunction with this minimal VB model yields an orientation of the anisotropy axis, which compares remarkably well with that obtained via rigorous ab initio calculations ( Table 1 ). To exemplify this correlation, we have calculated the magnetic properties of 14 low-symmetry monometallic dysprosium(III) complexes using the CASSCF ab initio methodology (see Methods) and compare them directly with our electrostatic model. In this work, we focus on the determination of magnetic anisotropy in cases of low symmetry. In high symmetry, the orientation of the ground Kramers doublet is pre-determined; note that in this case if V CF ( θ , ϕ ) does not stabilize the electron density along the symmetry axis, then m J =± 15 / 2 will not be the ground state. There is no such restriction in low-symmetry environments. Table 1 Comparison of ab initio and electrostatic calculations for Dy III complexes. Full size table Monometallic complexes The energy spectra and g -tensors of the ground 6 H 15/2 multiplets for compounds 1 – 14 , as calculated ab initio , are given in Supplementary Tables S1–S18 . Table 1 presents, for each complex, the principal value of the diagonal g -tensor of the ground Kramers doublet ( g z ) and the electrostatic deviation angle, defined as the angle between the electrostatic anisotropy axis and the ab initio anisotropy axis along which g z is defined. We note that the anisotropy axis is accurately predicted by employing this minimal VB model, without taking into account different electron withdrawing or donating groups in the charged ligands, for example, hfac − will have less electron density at the oxygen donor atoms compared with acac − because of the electron withdrawing nature of the CF 3 groups in the former ligand. Polymetallic complexes Calculating the ab initio properties of the following polymetallic complexes is extremely computationally expensive. Hence, to demonstrate the power of our simple approach, we have performed a semi-quantitative comparison between the electrostatic calculations and published ab initio results for three compounds: [Dy(MeCp) 2 (Ph 3 SiS)] 2 15 (ref. 28 ) [Dy 6 (teaH) 6 (NO 3 ) 6 ] 16 (refs 30 , 31 ) and [Dy 5 O( i PrO) 13 ] 17 (refs 32 , 33 ). The methodology for the calculation of the electrostatic anisotropy axes in polymetallic complexes is identical to that of monometallic complexes and is performed for each Dy III ion independently. The Dy III ions that are not the focus of the calculation are treated as part of the ligand and are given a +3 charge. The charged ligands in complexes 15 – 17 are given in Fig. 1 , which describes the charge partitioning based on the minimal VB model. The form of the potential (equation (2)) contains terms of for each charged atom in the ligand, which implies that the closer to the Dy III ion and larger the magnitude of the charge, the greater its effect on the orientation of the anisotropy axis. Complexes 1 – 9 contain three β-diketonate ligands in a ‘paddle-wheel’-like arrangement, with two β-diketonate ligands trans - to each other and the third trans- to a neutral ligand ( Fig. 2a ). If the quantization axis of the electron density was along the ‘paddle-wheel’ axis, then the radial plane of the approximately ‘oblate’ density would be coincident with all three charged ligands, representing a high-energy orientation. Therefore, the anisotropy axis is perpendicular to the ‘paddle-wheel’ axis, and we find that it passes through the two trans- β-diketonate ligands. The radial plane of the oblate electron density is thus coincident with only one charged ligand as opposed to two ( Fig. 2b and Supplementary Figs S1–S8 ). 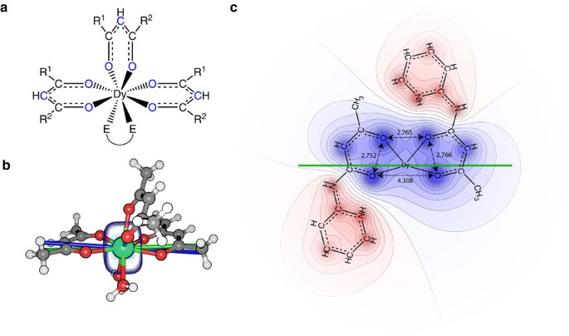Figure 2: Magnetic anisotropy and electrostatic potential of β-diketonate species. (a) Idealized ‘paddle-wheel’ geometry of complexes1–9viewed down the ‘paddle-wheel axis’. (b) Comparison of theab initio(blue rod) and electrostatic (green rod) anisotropy axes for the ground Kramers doublet in1, with the form of the oblatef-electron density using the representation of Sievers21, magnified approximately × 5 for clarity; Dy=green, O=red, C=grey and H=white. (c) Idealized electrostatic potential generated by a pair of paaH* ligands in the trapezium-shaped coordination environment present in the bis-β-diketonate-dysprosium(III) plane of compounds10and11and the resultant anisotropy axis (green line); red=positive potential, blue=negative potential. Figure 2: Magnetic anisotropy and electrostatic potential of β-diketonate species. ( a ) Idealized ‘paddle-wheel’ geometry of complexes 1 – 9 viewed down the ‘paddle-wheel axis’. ( b ) Comparison of the ab initio (blue rod) and electrostatic (green rod) anisotropy axes for the ground Kramers doublet in 1 , with the form of the oblate f-electron density using the representation of Sievers [21] , magnified approximately × 5 for clarity; Dy=green, O=red, C=grey and H=white. ( c ) Idealized electrostatic potential generated by a pair of paaH* ligands in the trapezium-shaped coordination environment present in the bis-β-diketonate-dysprosium(III) plane of compounds 10 and 11 and the resultant anisotropy axis (green line); red=positive potential, blue=negative potential. Full size image For compound 10 , the negatively charged oxygen atoms of the two β-diketonate ligands are the closest to Dy III and therefore have the greatest effect on the orientation of the anisotropy axis. These four atoms are roughly coplanar with the dysprosium(III) ion and are arranged in a trapezium ( Fig. 2c ). The oblate electron density will be in a high-energy configuration when the quantization axis is normal to this plane of four negative charges, and therefore the minimum electrostatic energy and anisotropy axis will lie in the plane of the β-diketonate oxygen atoms. The Dy III ion is much closer to the base of the trapezium and therefore if the quantization axis was to bisect the two parallel edges, then the radial plane of the electron density would interact strongly with the two basal oxygen atoms. If, however, the quantization axis was parallel with the base and top of the trapezium, there would be less interaction with the negative charges thus stabilizing the orientation. This is the orientation of the anisotropy axis ( Fig. 2c and Supplementary Fig. S9 ) calculated by our electrostatic model and it provides a simple explanation for the ab initio results. Analogous arguments can be made for compound 11 where the β-diketonate oxygen donors are in a similar trapezium-shaped arrangement, however, the coordination environment now contains two chelating nitrate anions. The oxygen atoms in NO 3 − have a larger negative partial charge than those in the β-diketonates, but this is offset by the positive charge on the nitrogen atom, which has an attractive effect on the electron density. Therefore, more-or-less the same anisotropy axis as in compound 10 is observed for compound 11 , along the diketonate-diketonate vector ( Supplementary Fig. S10 ). Compounds 1 – 10 have distorted square anti-prismatic geometries and the calculated anisotropy axis of the ground state is not found to be coincident with the pseudo-fourfold axis. This observation, shown here to be due to simple electrostatic arguments, is contrary to many reports in the literature that employ a fourfold axial interpretation to model the magnetic data (refs 25 , 34 , 35 , 36 ). Clearly, in these cases, the electrostatics are more important than pseudo-symmetry. Compounds 12 and 13 , chosen as a departure from β-diketonate-based complexes in addition to their very interesting magnetic properties, are intimately related and can be interconverted reversibly by drying or soaking in methanol, via a single crystal to single crystal transformation [7] . The difference between the dysprosium(III) coordination environments is the removal of a terminal methanol molecule, changing the local symmetry from a distorted pentagonal bipyramid to a distorted octahedron. Considering the local Dy III coordination environment, a pair of trans- phenoxo oxygen atoms in both 12 and 13 have much shorter Dy–O bond lengths than all others, at 2.21(2) Å compared with 2.39(2) Å for 12 and 2.186(4) Å compared with 2.3(1) Å for 13 , thus defining both geometries as axially compressed. In both cases, the three metal atoms are roughly coplanar with the equatorial planes of the coordination polyhedra. The close oxygen atoms define an axially repulsive potential for dysprosium(III), which, coupled with the attractive nature of the Zn 2+ cations in the equatorial plane, explains the observed magnetic anisotropy axes ( Supplementary Figs S11 and S12 ). In [Dy(DOTA)(H 2 O)Na 3 ] 2+ 14 , for which the magnetic anisotropy axis has been determined experimentally, the dysprosium(III) ion is encapsulated by the macrocyclic DOTA 4− ligand (ref. 37 ). The H atoms of the apical water molecule were not found experimentally, so were placed in calculated positions based on crystallographically characterized water molecules bound to Ln III ions (ref. 20 ). If the anisotropy axis was coincident with the pseudo -tetragonal axis, the radial plane of the oblate electron density would have a large interaction with the four negatively charged acetate groups, yielding a high-energy configuration ( Fig. 3a ). Therefore, the anisotropy axis is perpendicular to the pseudo -tetragonal axis of the molecule. The radial plane of the ‘oblate’ density is attracted by two Na + ions more strongly than just a single Na + ion ( Fig. 3b ), thus determining the observed orientation of the anisotropy axis ( Fig. 3c ), which agrees well with the experimentally determined and ab initio axes ( Table 1 ). We have rotated the apical water molecule in the ab initio calculations and found no dependence on the orientation of the ground state anisotropy axis to this perturbation, contrary to ref. 14 . 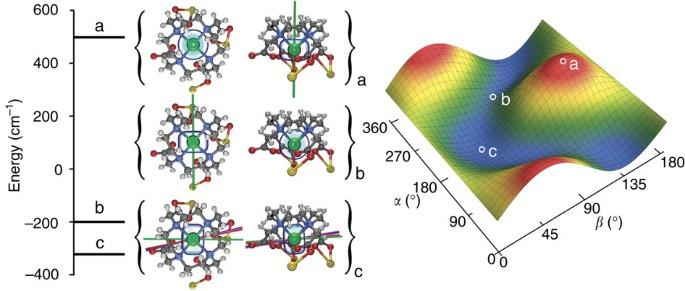Figure 3: Orthogonal configurations for the magnetic anisotropy axis in compound 14. The form of the oblatef-electron density, visualized in the central structural diagrams, follows the representation of Sievers21, and has been magnified approximately × 5 for clarity; Dy=green, Na=yellow, O=red, N=blue, C=grey and H=white. The rods in the central structural diagrams represent the magnetic anisotropy axes, identified by various methods: green=electrostatic calculation, dark blue=ab initiocalculation (this work), light blue=ab initiocalculation14and pink=experimentally determined. The energies of each configuration have been calculated using our electrostatic approach. The electrostatic energy surface is calculated by considering all possible orientations (α,β) of the anisotropy axis in the potential generated by the charged ligands of compound14. The electrostatic energy surface shows double degeneracy of the minimum, maximum and saddle points due to the axial symmetry of theelectron density. Figure 3: Orthogonal configurations for the magnetic anisotropy axis in compound 14. The form of the oblate f-electron density, visualized in the central structural diagrams, follows the representation of Sievers [21] , and has been magnified approximately × 5 for clarity; Dy=green, Na=yellow, O=red, N=blue, C=grey and H=white. The rods in the central structural diagrams represent the magnetic anisotropy axes, identified by various methods: green=electrostatic calculation, dark blue= ab initio calculation (this work), light blue= ab initio calculation [14] and pink=experimentally determined. The energies of each configuration have been calculated using our electrostatic approach. The electrostatic energy surface is calculated by considering all possible orientations ( α , β ) of the anisotropy axis in the potential generated by the charged ligands of compound 14 . The electrostatic energy surface shows double degeneracy of the minimum, maximum and saddle points due to the axial symmetry of the electron density. Full size image Compound 15 contains two dysprosium(III) ions bridged by two anionic Ph 3 SiS − ligands and each capped by two classical organometallic ligands, MeCp − (ref. 28 ). The two ions are related by inversion symmetry and therefore possess the same single-ion electronic structure. The electrostatic potential at each paramagnetic ion is dominated by the two MeCp − ligands, which are closer to the Dy III ion than the sulfur atoms at 2.65(3) Å (average Dy–C distance) compared with 2.76(2) Å. This leads to the anisotropy axis of the ground state lying perpendicular to the Dy-S-S-Dy plane ( Supplementary Fig. S13 ), in good agreement with ab initio calculations (ref. 28 ). The hexametallic dysprosium(III) wheel ( 16 ) contains highly anisotropic paramagnetic centres, yet due to crystallographic S 6 symmetry, possesses a diamagnetic ground state with a toroidal moment. Each Dy III ion is encapsulated by the teaH 2− ligand and also has one chelating nitrate anion [30] . Applying our electrostatic model to this compound yields the anisotropy axis of each dysprosium(III) site in excellent agreement with the ab initio results ( Supplementary Fig. S14 ) [31] . The anisotropy axis for each Dy III ion is canted around the ring in an alternating up/down manner, which, due to the S 6 symmetry of the molecule, causes the net cancellation of the out-of-plane magnetization in the ground state [31] , leading to a toroidal moment [8] , similar to that observed in a Dy 3 triangle [9] , [10] . It is remarkable that such a simple electrostatic approach can rationalize such complex physics. Compound 17 , with one of the highest energy barriers to the reversal of the ground state magnetization, contains five dysprosium(III) ions arranged in a pyramid, with each Dy III ion at the centre of an axially compressed octahedron. The equatorial plane of each ion is formed by four bridging isopropoxide ( i PrO − ) ligands and the axial positions are occupied by the single μ 5 -oxide bridge at the centre of the molecule and a terminal isopropoxide ligand [32] . The oxygen atom of the terminal i PrO − ligand is substantially closer to the Dy III ion than all other donor atoms, at 2.04(1) Å compared with 2.35(8) Å, and the central μ 5- oxide has a double negative charge. These two features define a strongly repulsive axial potential for the electron density, where the energy is minimized when the quantization axis is coincident with this direction ( Fig. 4 ). The presence of the other charged ligands and the trivalent dysprosium ions is a small perturbation in this case, because of the strongly directional nature of the almost linear i PrO − -Dy-O 2− axis. The results obtained using our electrostatic model compare extremely well with those obtained using ab initio calculations [33] (see Supplementary Table S19 ). 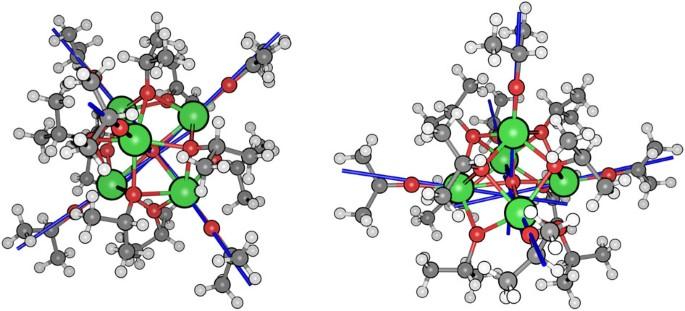Figure 4: Ground state magnetic anisotropy of compound 17. The blue rods represent the orientations of the anisotropy axes for each of the five DyIIIions in complex17as calculated by our electrostatic model; Dy=green, O=red, C=grey and H=white. Figure 4: Ground state magnetic anisotropy of compound 17. The blue rods represent the orientations of the anisotropy axes for each of the five Dy III ions in complex 17 as calculated by our electrostatic model; Dy=green, O=red, C=grey and H=white. Full size image Calculation of the ground state magnetic anisotropy axis of Dy III in low-symmetry environments, employing an electrostatic minimization strategy, shows how simple chemical intuition can aid in the understanding of a complex problem of electronic structure. Given the success of the electrostatic model in the cases presented, we propose that this model can be used to aid in the rational design of molecular architectures displaying novel magnetic properties, exploiting and stabilizing the strong axiality of the ground state of low-symmetry dysprosium(III), through the use of formally charged ligands. The simplicity of the proposal is so profound that the model resonates strongly with the conclusions drawn in the 1950s and 1960s that the bonding of the lanthanides is almost purely ionic (refs 38 , 39 ). By entirely neglecting the influence of neutral ligands in our model, we have shown the dominant nature of charged ligands in the determination of the magnetic anisotropy of dysprosium(III) complexes. Compounds lacking any charged ligands are rare, but would likely show magnetic anisotropies that are much more sensitive to the type of ligands present, with contributions due to dipoles and higher order multipoles as well as the spatial extent of ligand electron density becoming important. The minimal VB model for the partitioning of charges on ligands works well for the formally charged ligands presented here. Other more general schemes for the partitioning of atomic charges over the ligands are also being investigated, which may offer an improvement over the minimal VB model. We are also extending the method to other lanthanide ions, examining whether this approach can work for other oblate ions (for example, Tb III ) and whether the reverse electrostatic principles will apply to prolate ions (for example, Er III ). Although the treatment presented here cannot be rigorously applied to non-Kramers ions in low-symmetry environments, Tb III complexes that possess a pseudo -doublet ground state with m J = ±6 ( g x = g y =0, g z =18) should follow similar electrostatic arguments to those discussed here for the determination of the magnetic anisotropy. Conversely, preliminary results suggest that the ground state wavefunctions of Er III ions in low-symmetry environments are not well defined and consist of strongly mixed m J states, precluding the application of the treatment presented here. The work presented here is an advance not only for the chemistry and physics communities involved with molecular magnetism, but also for all areas concerned with the magnetic and spectroscopic properties of the lanthanides. Specifically, this work provides some much-needed insight into the complex and continually intriguing magnetic properties of dysprosium(III). High-level quantum chemical calculations such as CASSCF are computationally expensive and require intervention by experts to produce reliable results. The complementary approach we outline here is available to any chemist with minimal computational requirements. Electrostatic calculations The electrostatic calculations were performed on the complete monometallic structures (excluding lattice solvent or non-coordinated counter ions) using the reported X-ray geometry with no optimization. The charges were assigned to the ligands as described in the text and all other atoms did not contribute to the potential. The angles describing the orientation of the electron density with respect to the experimental geometry, ( α , β ), were then optimized to minimize the electrostatic energy. In applying this strategy, we have evaluated the uncertainty associated with using X-ray coordinates by moving the atomic positions by a random factor within the estimated standard deviations and found that the change in the orientation of the anisotropy axis over all monometallic compounds studied is on the order of 1°. We have elected to use the Freeman and Watson values for the average radial integrals (ref. 40 ), ‹ r k ›, and have investigated the effect of these values on the calculated anisotropy direction and also found deviations on the order of 1° when their values are altered non-systematically by up to 20%. The electrostatic calculations were implemented in a FORTRAN program, MAGELLAN, which is available from the authors upon request. Ab initio calculations CASSCF calculations were performed with MOLCAS 7.6 (refs 12 , 41 , 42 ) on the same geometry as used for the electrostatic calculations. The ANO-RCC-VTZP, VTZ and VDZ basis sets were used for the dysprosium ion, first coordination sphere atoms and all other atoms, respectively. The calculations employed the second order Douglas–Kroll–Hess Hamiltonian, where scalar relativistic contractions are taken into account in the basis set and the spin-orbit coupling is handled separately in the RASSI module. The active space for dysprosium was, in all cases, nine electrons in seven orbitals. It was found that the effect of the spin quartets and doublets was negligible on the orientation of the magnetic anisotropy and therefore only the 21 spin sextets were included in the state averaged CASSCF and spin-orbit coupling calculations. The effect of CASPT2 corrections for dynamic electron correlation were investigated, but found to have a minor role in the orientation of the magnetic anisotropy, where the extent of the basis set had much more of an impact, and therefore CASPT2 corrections were not performed. Cholesky decomposition of the two-electron integrals was performed to save disk space and computational time. These three approximations combined led to differences in the calculated ground state orientation for 1 of less than 1°, which is comparable with the uncertainty in the calculation of the electrostatic orientations, vide supra . How to cite this article: Chilton, N.F. et al. An electrostatic model for the determination of magnetic anisotropy in dysprosium complexes. Nat. Commun. 4:2551 doi: 10.1038/ncomms3551 (2013).